ArabidopsisWAT1 is a vacuolar auxin transport facilitator required for auxin homoeostasis The plant hormone auxin (indole-3-acetic acid, IAA) has a crucial role in plant development. Its spatiotemporal distribution is controlled by a combination of biosynthetic, metabolic and transport mechanisms. Four families of auxin transporters have been identified that mediate transport across the plasma or endoplasmic reticulum membrane. Here we report the discovery and the functional characterization of the first vacuolar auxin transporter. We demonstrate that WALLS ARE THIN1 (WAT1), a plant-specific protein that dictates secondary cell wall thickness of wood fibres, facilitates auxin export from isolated Arabidopsis vacuoles in yeast and in Xenopus oocytes. We unambiguously identify IAA and related metabolites in isolated Arabidopsis vacuoles, suggesting a key role for the vacuole in intracellular auxin homoeostasis. Moreover, local auxin application onto wat1 mutant stems restores fibre cell wall thickness. Our study provides new insight into the complexity of auxin transport in plants and a means to dissect auxin function during fibre differentiation. Auxin has a crucial role in multiple aspects of plant growth and development, from controlling plant architecture, directional growth responses and abiotic and biotic stress responses to regulating reproductive and vascular development [1] , [2] , [3] . Diffusion of auxin across membranes is limited and at least four distinct transporter families have evolved to facilitate intercellular and intracellular transport. The AUX1/LAX influx transporter protein family was originally found through the isolation of the Arabidopsis auxin resistant1 ( aux1 ) mutant. aux1 roots are resistant to the membrane impermeable synthetic auxin, 2,4-dichlorophenoxyacetic acid (2,4- D ), and show agravitropic growth as consequences of a defect in cellular auxin uptake. The AUX1 gene codes for a protein homologous to amino-acid permeases [4] that mediates auxin import when heterologously expressed in Xenopus laevis oocytes [5] . The second class of auxin transporters is represented by the ATP-binding cassette subfamily B (ABCB)-type transporters of the MULTIDRUG RESISTANCE/phosphoglycoprotein (ABCB/MDR/PGP) family of membrane proteins, which mediate ATP-dependent auxin transport through the plasma membrane [6] . ABCB1, ABCB4 and ABCB19 have been identified as proteins with binding affinity to the auxin transport inhibitor 1-naphthylphthalamic acid [6] , [7] . The biochemical evidence for these ABCB proteins having a role in auxin transport has been provided by heterologous expression in tobacco cells, HeLa cells and yeast [8] , [9] , [10] . Finally, PIN-FORMED (PIN) family members have a critical role in determining the directionality of auxin flow in embryonic and post-embryonic development [11] . In contrast to ABC transporters, which occur across all kingdoms, PIN genes are plant specific [12] . The canonical ‘long’ PIN proteins PIN1–4 and 7 are localized at the plasma membrane and ensure auxin efflux [13] . However, it was shown recently that PIN5 and PIN8, two atypical ‘short’ PINs with a shorter hydrophilic loop, are localized at the endoplasmic reticulum (ER) [14] , [15] , [16] , highlighting the importance of intracellular mechanisms in controlling auxin homoeostasis. Similarly, the PIN-LIKES (PILS) protein family has recently been identified based on in silico structural homology with PIN5. PILS proteins have been suggested to regulate intracellular auxin accumulation at the ER [17] . A gene expression profiling approach previously identified hundreds of candidate genes for secondary cell wall formation in Zinnia elegans xylogenic cell cultures [18] . Mutations in an Arabidopsis homologue of one of these genes, WALLS ARE THIN1 ( WAT1 ), caused a drastic reduction in secondary cell wall thickness of stem fibres [19] . The WAT1 protein is similar in sequence to a Medicago truncatula nodulin 21, originally shown to be upregulated in Rhizobium -induced Medicago nodules [20] . The Arabidopsis WAT1 gene family is composed of 46 members. WAT1 has been proposed to be involved in integrating auxin signalling and secondary cell wall formation in Arabidopsis fibres [19] based on transcriptomic, metabolomic and physiological data. The wat1-1 mutation resulted in the massive downregulation of auxin-related gene expression and reduced auxin content in stems, and an increased sensitivity of wat1 seedlings to 5-Methyl-Trp, a toxic analogue of Trp, an auxin precursor. In this study, we demonstrate that WAT1 is a so far unknown tonoplast-localized auxin transporter, suggesting a critical role for the vacuole in regulating intracellular auxin homoeostasis in plants. Further, the fact that the reduction in secondary cell wall thickenings in wat1 mutants can be rescued by exogenous auxin application underpins the role of auxin in secondary growth in plants. A link between WAT1 and auxin responses A microarray-wide search for the most highly co-regulated genes with WAT1 (ref. 21 ) resulted in the identification of several genes involved in auxin transport and signalling (that is, AUX1 , IAA9 , IAA13 , LAX2 , ARF4, ARF11 and PIN1 ; Fig. 1 ). Consistent with the cell wall phenotype of wat1 mutants, other WAT1 co-regulated genes are known to be essential for either vascular patterning ( ATHB-8 and ATHB-15 ) or secondary wall deposition ( IRX9 , MYB43 , KNAT7 and FRA1 ). Strikingly, the expression of several of these genes, including WAT1 itself, is also induced by auxin ( Figs 1 and 2 ). 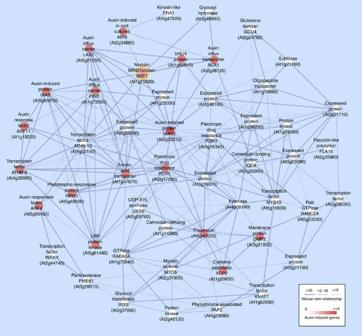Figure 1: WAT1 coexpression vicinity network. The most highly co-regulated genes withWAT1as identified with theArabidopsisCoexpression Data Mining Tools from the University of Leeds21(http://www.Arabidopsis.leeds.ac.uk/act/coexpanalyser.php). Nodes represent genes; edge width indicates whether two given genes are co-expressed above a certain mutual rank threshold56. Nodes are colour coded to reflect the level of induction by auxin of the corresponding genes according to the Genevestigator22(https://www.genevestigator.com) and the Bio-Array Resource57(http://www.bar.utoronto.ca) websites. Figure 1: WAT1 coexpression vicinity network. The most highly co-regulated genes with WAT1 as identified with the Arabidopsis Coexpression Data Mining Tools from the University of Leeds [21] ( http://www.Arabidopsis.leeds.ac.uk/act/coexpanalyser.php ). Nodes represent genes; edge width indicates whether two given genes are co-expressed above a certain mutual rank threshold [56] . Nodes are colour coded to reflect the level of induction by auxin of the corresponding genes according to the Genevestigator [22] ( https://www.genevestigator.com ) and the Bio-Array Resource [57] ( http://www.bar.utoronto.ca ) websites. 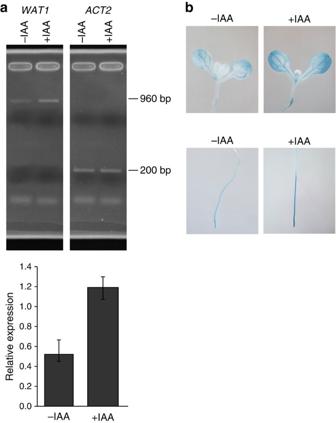Figure 2:WAT1is induced by auxin. (a) Reverse transcriptase (RT)–PCR analysis ofWAT1expression in 10-day-old wild-type plantlets transferred for 2 h on MS medium with or without 1 μM IAA before RNA extraction. The amount of cDNA template in each RT–PCR reaction was normalized to the signal from the actin-encodingACT2gene, and primers were designed to rule out the amplification of genomic DNA. Histograms representWAT1expression levels normalized versusACT2expression levels. Mean±s.d.,n=3 biological replicates. (b) GUS activity in the aerial portion (top) and roots (bottom) of 10-day-old ProWAT1:GUSplantlets transferred for 2 h on MS medium with or without 1 μM IAA before staining. Full size image Figure 2: WAT1 is induced by auxin. ( a ) Reverse transcriptase (RT)–PCR analysis of WAT1 expression in 10-day-old wild-type plantlets transferred for 2 h on MS medium with or without 1 μM IAA before RNA extraction. The amount of cDNA template in each RT–PCR reaction was normalized to the signal from the actin-encoding ACT2 gene, and primers were designed to rule out the amplification of genomic DNA. Histograms represent WAT1 expression levels normalized versus ACT2 expression levels. Mean±s.d., n =3 biological replicates. ( b ) GUS activity in the aerial portion (top) and roots (bottom) of 10-day-old Pro WAT1 : GUS plantlets transferred for 2 h on MS medium with or without 1 μM IAA before staining. Full size image Phenotypic alterations resulting from the wat1 mutation have been reported at late stages of plant stem development; however, WAT1 is expressed much earlier in plant development [19] ( Fig. 2 ). To elucidate primary effects of the wat1 mutation, we carried out comparative microarray analysis profiling mRNA global expression of 10-day-old in vitro -grown wild-type and wat1-1 -mutant seedlings. This revealed 40 genes that exhibited significantly altered expression levels in wat1-1, with 13 genes displaying lower and 27 higher mRNA levels compared with the wild type ( Supplementary Fig. S1 ). The two most downregulated genes, besides WAT1 itself, were IAA19 and an auxin-responsive GH3 family member both known to be associated with auxin responses. Among the 13 downregulated genes, at least 7 are induced by auxin in wild-type plants according to the Genevestigator database [22] ( Supplementary Fig. S1 ). In contrast, among the 27 genes upregulated in wat1 , 5 are repressed by auxin in wild-type plants ( Supplementary Fig. S1 ). These results revealed that the wat1-1 mutation modulates the expression levels of several auxin-responsive genes. Finally, to determine whether there is a causal link between lower auxin content and the fibre phenotype in wat1 stems [19] , we locally applied auxin (2,4- D and NAA) to growing stem segments of wat1 . Ten days after auxin application, cell wall thickness of wat1 interfascicular fibres was restored to wild-type levels ( Fig. 3 ). These results confirm the role of auxin in promoting xylem fibre differentiation [23] , [24] . 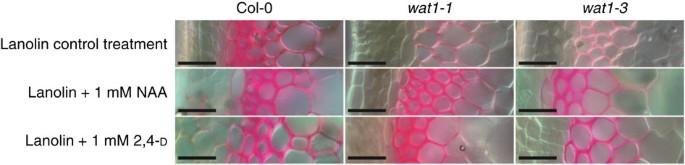Figure 3:Local auxin application rescues deficiency in secondary cell wall formation inwat1mutants. Phloroglucinol-HCl staining of transverse stem sections, lignified cell walls stained red. Lanolin±auxin was applied to the second oldest internode of the inflorescence stem. Stems were sectioned 10 days after application. Sections are representative of data from two experimental replicates each with six individuals per genotype and treatment. Scale bars, 50 μm. Figure 3: Local auxin application rescues deficiency in secondary cell wall formation in wat1 mutants. Phloroglucinol-HCl staining of transverse stem sections, lignified cell walls stained red. Lanolin±auxin was applied to the second oldest internode of the inflorescence stem. Stems were sectioned 10 days after application. Sections are representative of data from two experimental replicates each with six individuals per genotype and treatment. Scale bars, 50 μm. Full size image WAT1 is a tonoplast-localized auxin transporter The WAT1 gene encodes a plant-specific protein of 389 amino acids [19] predicted to have 10 transmembrane domains, and it has been classified as a member of the Plant Drug Metabolite Exporter family (Transport Classification Database ( http://www.tcdb.org ) [25] , [26] ). Although PINs and AUX1 are members of the auxin efflux carrier and amino acid/auxin permease families, respectively, several of them also possess 10 predicted transmembrane domain. Although WAT1 did not exhibit sequence homology with any of the other auxin transporters, its predicted secondary structure was similar, showing the greatest resemblance with the ER-localized PIN5 and PILS2/5 proteins ( Supplementary Fig. S2 ). Beyond their similarity in size, they have a centrally localized, shorter hydrophilic loop in comparison with the ‘long PINs’ (PIN1–4, 7). Although WAT1 has been previously detected in both plasma membrane and tonoplast fractions in systematic proteomic studies [27] , [28] , we found very little co-localization of WAT1-GFP (green fluorescent protein) with the plasma membrane marker, yellow fluorescent protein (YFP)-NPSN12 (ref. 29 ) ( Fig. 4a ). In contrast, WAT1-GFP co-localized to the greatest extent with the tonoplast marker, YFP-VAMP711 ( Fig. 4a ), consistent with our previous interpretation that WAT1 may be a tonoplast-localized protein [19] . WAT1-GFP exhibited some overlapping fluorescent signal with the late endosomal marker, YFP-RabG3f, but to a lesser extent than with YFP-VAMP711. As in the case for the tonoplast marker YFP-VAMP711, WAT1-GFP localization was also insensitive to Brefeldin A (BFA) treatment ( Supplementary Fig. S3 ), suggesting that WAT1-GFP was delivered to the tonoplast by a BFA-insensitive, Golgi-independent pathway [30] . 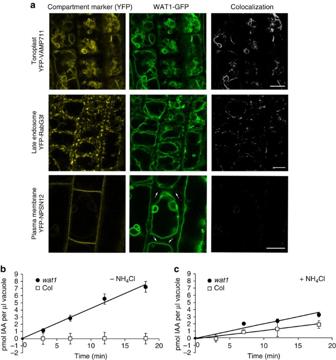Figure 4: WAT1 is a vacuolar auxin transporter. (a) Co-localization of WAT1-GFP with known fluorescent membrane markers. F1 generation of crosses betweenp35S::WAT1-GFPand plants expressing either YFP-VAM711, a tonoplast marker (top row), YFP-RabG3f, a late endosome marker (central row) or YFP-NPSN12, a plasma membrane marker (bottom row). Co-localization in root epidermis cells in the elongation zone of 5-day-oldArabidopsisseedlings is shown. Note strong co-localization of WAT1-GFP with the tonoplast marker, partial co-localization with the late endosome marker and weak co-localization with the plasma membrane marker. Weak signal of WAT1-GFP at the plasma membrane (arrows). Scale bars, 10 μm. (b), Time-dependent transport of auxin in vacuoles isolated from wild-type plants andwat1mutants in the absence of NH4Cl. The values represent means of five replicates, and the error bars stand for ±s.e.m. Simplified transport experiments with five replicates each at short and long time points were performed four times; their outcome is in line with the extended time course experiment. (c) Same asb, except in the presence of NH4Cl and the omission of Mg-ATP. Figure 4: WAT1 is a vacuolar auxin transporter. ( a ) Co-localization of WAT1-GFP with known fluorescent membrane markers. F1 generation of crosses between p35S::WAT1-GFP and plants expressing either YFP-VAM711, a tonoplast marker (top row), YFP-RabG3f, a late endosome marker (central row) or YFP-NPSN12, a plasma membrane marker (bottom row). Co-localization in root epidermis cells in the elongation zone of 5-day-old Arabidopsis seedlings is shown. Note strong co-localization of WAT1-GFP with the tonoplast marker, partial co-localization with the late endosome marker and weak co-localization with the plasma membrane marker. Weak signal of WAT1-GFP at the plasma membrane (arrows). Scale bars, 10 μm. ( b ), Time-dependent transport of auxin in vacuoles isolated from wild-type plants and wat1 mutants in the absence of NH 4 Cl. The values represent means of five replicates, and the error bars stand for ±s.e.m. Simplified transport experiments with five replicates each at short and long time points were performed four times; their outcome is in line with the extended time course experiment. ( c ) Same as b , except in the presence of NH 4 Cl and the omission of Mg-ATP. Full size image The subcellular localization of WAT1 and its structural resemblance to auxin carriers prompted us to test the capacity of WAT1 to transport indole-3-acetic acid (IAA) across the tonoplast membrane. Therefore, we isolated vacuoles from wat1 and wild-type mesophyll protoplasts and carried out transport studies using 14 C-IAA. Experiments were conducted at pH 7.6, a condition under which IAA is present mainly in the anionic, unprotonated form, and diffusion is minimal. As a control, 3 H 2 O was added to the incubation medium as water readily diffuses through biological membranes. This confirmed the volume, intactness and stability of both wild-type and wat1 vacuole populations. Auxin did not accumulate in wild-type vacuoles, whereas in wat1 vacuoles, the auxin concentration increased in a time-dependent manner ( Fig. 4b ). If we assume that auxin uptake rates are similar in both vacuole populations, this points to an efficient, WAT1-dependent auxin efflux from wild-type vacuoles, which is obviously absent in wat1 vacuoles. As exporting anionic auxin from the vacuole is thermodynamically uphill, a likely energy source would be the coupling with downhill transport of protons (for a review, see ref. 31 ). Therefore, we hypothesize that WAT1 is a tonoplast-localized transporter that exports auxin from the vacuole to the cytoplasm, perhaps operating as a H + :IAA − symporter. To test this hypothesis, additional vacuole transport experiments were performed under conditions that ensured a drastic reduction of the driving force for proton-coupled exporters ( Fig. 4c ). NH 4 + , a proton gradient dissipater, was added to the external buffer, whereas Mg-ATP was omitted to avoid compensation of proton gradient dissipation by V-ATPase-mediated proton pumping into the vacuole. In this experiment, NH 4 + should theoretically reduce IAA efflux from wild-type vacuoles, resulting in a net increase in vacuolar IAA concentration over time. This was the case ( Fig. 4c ), thereby supporting the hypothesis that WAT1 operates as a H + -IAA − symporter. In the presence of NH 4 + and absence of Mg-ATP, not only is the pH gradient expected to decrease but also the difference in electrical potential across the tonoplast, which is a driving force for IAA − uptake. This explains the decrease in IAA accumulation in wat1 vacuoles in the presence of NH 4 + (absence of Mg-ATP; Fig. 4c ) versus the absence of NH 4 + and presence of Mg-ATP ( Fig. 4b ). It is noteworthy that the reduced difference in membrane potentials should lead to a similar reduction of IAA influx towards the vacuole lumen in wild type. The fact that a net increase of IAA levels in wild-type vacuoles in the presence of NH 4 + was observed strengthens our conclusion that WAT1 efflux was primarily affected by NH 4 + application. Finally, to determine whether the radiolabelled 14 C detected during vacuolar transport experiments was uniquely associated with IAA or converted to other related metabolites, high performance liquid chromatography (HPLC) analysis was performed on wild-type vacuoles. Only one major peak corresponding to IAA was detected, confirming that the radiolabel was associated uniquely to IAA ( Fig. 5 ). Altogether, these results strongly support the hypothesis that WAT1 mediates IAA export from the vacuole. 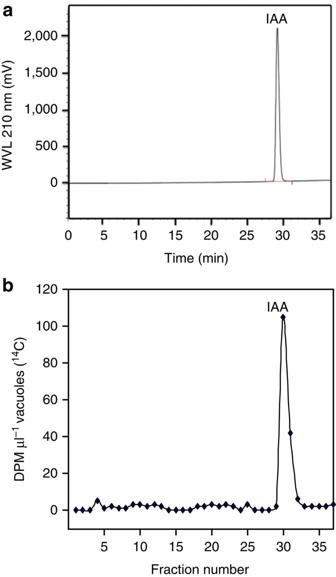Figure 5: Auxin fractionation after vacuole uptake. Auxin is not converted within vacuoles. Isolated vacuoles were incubated in the presence of14C-auxin (IAA) for 20 min and subsequently removed from the incubation medium as described for the transport studies. The water phase containing the vacuoles was subjected to a HPLC run, fractions were collected and the radioactivity present in each fraction was detected. A comparison of panela, where non-radioactive auxin was detected at 29 min, with panelbrepresenting the radioactivity detected in each fraction, shows that the radioactivity appears at a similar retention time as the authentic auxin. The slight shift is because of the collection of the fractions that occurred after the ultraviolet detector. WVL, wavelength. For more details see Methods. Figure 5: Auxin fractionation after vacuole uptake. Auxin is not converted within vacuoles. Isolated vacuoles were incubated in the presence of 14 C-auxin (IAA) for 20 min and subsequently removed from the incubation medium as described for the transport studies. The water phase containing the vacuoles was subjected to a HPLC run, fractions were collected and the radioactivity present in each fraction was detected. A comparison of panel a , where non-radioactive auxin was detected at 29 min, with panel b representing the radioactivity detected in each fraction, shows that the radioactivity appears at a similar retention time as the authentic auxin. The slight shift is because of the collection of the fractions that occurred after the ultraviolet detector. WVL, wavelength. For more details see Methods. Full size image These findings raised the question as to whether auxin is actually present in plant vacuoles. Although early physiological studies in the green alga Hydrodictyon [32] speculated that the vacuole of higher plants might represent a pool of symplastic auxin [33] , experimental evidence for vacuolar auxin in plants is still lacking. To address whether auxin is found in Arabidopsis vacuoles, vacuoles were purified from protoplasts of wild-type leaves and IAA and related metabolites were measured ( Table 1 ). Vacuole purity was first confirmed by western blots using antibodies detecting different cellular compartment markers ( Supplementary Fig. S4 ). Strikingly, IAA, several of its precursors, the IAA catabolite oxIAA (oxIAA) and the conjugate IAA-Glc could be detected in purified vacuoles ( Table 1 ), suggesting an important role for the vacuole in auxin storage and regulation of auxin homoeostasis in Arabidopsis . The apparent discrepancy in our observations that auxin and related metabolites were found in isolated vacuoles while isolated wild-type vacuoles did not take up auxin in transport experiments ( Fig. 4b ) suggests that WAT1 can act as an efficient auxin exporter but that its activity is likely regulated in vivo. Table 1 IAA and related metabolite content in wild-type vacuoles. Full size table WAT1 auxin transport activity in yeast and Xenopus oocytes To confirm WAT1 auxin transport activity, we cloned the complementary DNA of WAT1 into the yeast expression vector pDR196 and introduced it into Saccharomyces cerevisiae . As demonstrated by reverse transcriptase–PCR, WAT1 was highly expressed in yeast transformed with pDR196- WAT1 ( Fig. 6a ). When fused with GFP, WAT1 localized to the plasma membrane of yeast cells ( Fig. 6b ). WAT1 expression resulted in a significant increase in radiolabelled 3 H-IAA uptake as compared with the empty vector control ( Fig. 6c ). The specificity of IAA transport was confirmed by performing 3 H-IAA transport in the presence of various non-radioactive potential competitors ( Fig. 6d ). 3 H-IAA influx in yeast expressing WAT1 was greatly inhibited by unlabelled IAA (69%) and to a lesser degree (25% and 27%) by oxIAA and 1-naphthaleneacetic acid (NAA), respectively. Conjugated forms of IAA (IAA- L -alanine, IAA- L -phenylalanine and IAA-Glc) and other forms of natural or synthetic auxinic compounds (indole-3-butyric acid and 2,4- D ) did not reduce WAT1-mediated 3 H-IAA influx in yeast. Finally, WAT1 did not facilitate 3 H-Trp uptake ( Fig. 6e ). WAT1-mediated IAA influx was further confirmed by testing it in an independent heterologous expression system: Xenopus oocytes ( Fig. 6f ). As compared with water-injected oocytes, WAT1 complementary ribonucleic acid (cRNA)-injected oocytes incorporated significantly more 3 H-IAA. WAT1 did not facilitate Trp import or export in oocytes: influx and efflux of 15 N-labelled Trp in WAT1-expressing oocytes were 100.02%±0.13 ( n =11) and 101.13%±1.09 ( n =8) that of control oocytes, respectively (mean±s.d.). These data confirm that WAT1 catalyses a net influx of IAA, in agreement with data obtained in yeast. These results demonstrate that WAT1-mediated IAA transport activity does not require any additional, plant-specific components. 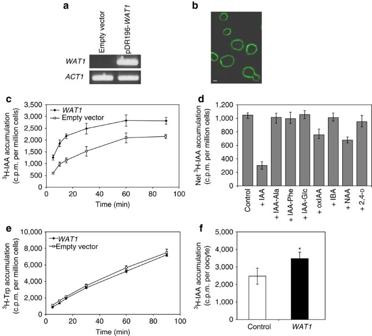Figure 6:WAT1 confers auxin efflux to yeast cells andXenopusoocytes. (a)WAT1transcript levels in yeast transformed either with the empty pDR196 vector or with pDR196-WAT1. Actin (ACT1) primers were used as control. (b) Subcellular localization in yeast of GFP-tagged WAT1. Scale bar, 1 μm. (c)3H-IAA transport assay in yeast. Closed circles, yeasts expressing WAT1; open squares, control yeasts containing the empty vector. Mean±s.d.,n=3 biological replicates. (d) Net accumulation in 15 min of3H-IAA in WAT1-expressing yeast (relatively to control yeast containing the empty vector) in the presence of 500 μM potential non-radiolabelled competitors. Mean±s.d.,n=3 biological replicates. (e)3H-tryptophan transport assay in yeast. Same asc. (f) Expression ofWAT1increases auxin uptake inXenopusoocytes. Auxin uptake was measured by the incorporation of3H-labelled IAA (see Methods). Data are displayed as mean values (±s.d.) of auxin influx in oocytes injected either with deionized water (‘control’,n=10) or withWAT1cRNAs (‘WAT1’,n=10). *, a Student’s test (threshold 0.98) showed that ‘WAT1’ mean value is statistically different from the ‘control’. Figure 6: WAT1 confers auxin efflux to yeast cells and Xenopus oocytes. ( a ) WAT1 transcript levels in yeast transformed either with the empty pDR196 vector or with pDR196- WAT1 . Actin ( ACT1 ) primers were used as control. ( b ) Subcellular localization in yeast of GFP-tagged WAT1. Scale bar, 1 μm. ( c ) 3 H-IAA transport assay in yeast. Closed circles, yeasts expressing WAT1; open squares, control yeasts containing the empty vector. Mean±s.d., n =3 biological replicates. ( d ) Net accumulation in 15 min of 3 H-IAA in WAT1-expressing yeast (relatively to control yeast containing the empty vector) in the presence of 500 μM potential non-radiolabelled competitors. Mean±s.d., n =3 biological replicates. ( e ) 3 H-tryptophan transport assay in yeast. Same as c . ( f ) Expression of WAT1 increases auxin uptake in Xenopus oocytes. Auxin uptake was measured by the incorporation of 3 H-labelled IAA (see Methods). Data are displayed as mean values (±s.d.) of auxin influx in oocytes injected either with deionized water (‘control’, n =10) or with WAT1 cRNAs (‘WAT1’, n =10). *, a Student’s test (threshold 0.98) showed that ‘WAT1’ mean value is statistically different from the ‘control’. Full size image It is important to note that transporters maintain their orientation with respect to the cytoplasm so that protein domains facing the cytoplasm in the native context also face the cytoplasm in these heterologous expression systems. Therefore, if the thermodynamic conditions are favourable, they also maintain their direction of transport (with respect to the cytosol) when targeted to a different membrane in heterologous expression systems (in this case, the plasma membrane as opposed to the tonoplast) [14] , [34] . The conditions used in our heterologous expression systems are compatible with the thermodynamics between the cytosol and vacuole. Therefore, WAT1-mediated IAA import from the medium towards the cytosol in yeast and oocytes would correspond to vacuolar export towards the cytosol (equivalent to the external solution in isolated vacuoles experiments).Therefore, yeast and oocyte IAA transport data both independently confirm that WAT1 acts as an auxin exporter in vacuoles. Herein we demonstrate that Arabidopsis thaliana WAT1 encodes a novel auxin transporter in plants. Although WAT1 is already expressed during seed germination and seedling development, the wat1 phenotype only becomes apparent at later stages of plant development. We show that the most conspicuous phenotype, a decrease in stem fibre cell wall thickness [19] , could be restored by exogenous auxin application to stems. Mutations in the class III HD ZIP transcription factor REVOLUTA also led to impaired fibre differentiation, and this phenotype was correlated with reduced expression of several PIN genes and reduced polar auxin transport [24] . However, the discovery that WAT1 possesses auxin transport activity and that the fibre phenotype in wat1 mutants can be restored by exogenous application of auxin provide the first direct genetic evidence for a role of auxin in fibre differentiation. As vacuole-localized auxin cannot bind to nuclear or ER-localized auxin receptors, active redirection of vacuolar auxin to the cytoplasm might be critical for auxin signalling, especially in strongly vacuolated cells such as interfascicular fibres. Despite the absence of a seedling phenotype, a mutation in WAT1 altered the expression of several auxin-regulated genes. As free auxin content in wat1 seedlings is similar to wild type [19] , the deregulation of auxin-related genes may be due to wat1 -mediated changes in the subcellular compartmentation of auxin. The regulation of auxin homoeostasis via intracellular compartmentalization is becoming an increasingly central theme in auxin biology [35] , [36] . The role of the ER in auxin metabolism and signalling had already been inferred by the presence of auxin-binding protein 1 (ABP1), an auxin receptor involved in determining cell expansion rate [37] , gene expression [38] , Rho-GTPase-dependent cytoskeleton organization [39] , and clathrin-dependent endocytosis [40] and of IAA–amino acid amidohydrolases in the ER lumen [41] . The recent discovery that PIN5 and PIN8, two atypical members of the PIN family, mediate auxin flow between the cytosol and ER lumen further reinforces the major role of the ER in auxin homoeostasis [14] , [15] , [16] . It has recently been postulated that PIN5 residence/activity at the ER is regulated by ABP1 in a similar manner that extracellular ABP1 regulates PIN protein activity at the PM [35] , [40] . The similarities between WAT1, PIN5 and PILS2/5 are striking; the predicted proteins bear structural resemblance to one other and from a functional standpoint, they mediate intracellular auxin homoeostasis. These features, along with the fact that they all have homologues in basal land plants [42] , [43] suggest an ancient, conserved, auxin transporter structure and support the theory that intracellular regulation of auxin metabolism is an ancient event in the evolution of land plants [44] . To our knowledge, this is the first report demonstrating a role for the vacuole in the regulation of auxin homoeostasis. WAT1-mediated auxin transport across the tonoplast membrane uncovers an additional level of intracellular complexity in auxin signalling pathways in plant cells. Paradoxically, the presence of auxin and its metabolites in vacuoles has never been demonstrated, although in earlier physiological studies it has been inferred [32] , [33] . 14 C-IAA transport assays carried out on isolated vacuoles showed that WAT1 exports IAA from the vacuole to the external medium, the equivalent to the cytoplasm in plant cells. This directionality is strongly supported by the overall decrease in auxin response gene expression in wat1 seedlings and heterologous expression data in yeast, whereby WAT1 facilitates auxin uptake from the extracytoplasmic space into the cytosol. Most vacuolar transporters use an electrochemical gradient and act either as vacuolar proton antiporters for import processes or proton symporters to export compounds [31] . H + -V-ATPases and H + -PPases generate a trans -tonoplast H + electrochemical gradient, with a positive electrical potential and a lower pH in the vacuole with respect to the cytosol or external medium [31] . In Arabidopsis , the vacuolar pH is around 6. This means that vacuolar auxin is essentially in the non-permeant, anionic form and its export would be thermodynamically uphill. As WAT1-mediated auxin export required energy in isolated vacuole transport experiments, this is also likely to be the case in vivo . Although it is clear that PINs, PILS, ABCBs, AUX-LAXs proteins and now WAT1 are essential factors in auxin transport, there are clearly other potential candidates within plant genomes. Of the 25,498 predicted proteins in the Arabidopsis genome, 5–10% are thought to be transporters [45] , and among them, only a limited number has been assigned a biological function. Some transporters might even transport several substrates. One example is the previously characterized NRT1.1 nitrate transporter, which is also capable of transporting auxin at low nitrate concentrations [46] . Although we cannot categorically exclude that WAT1 might also be multifunctional, our results clearly demonstrate its capacity to facilitate auxin transport, and the fact that the wat1 phenotype can be rescued by applying auxin supports its major role as an auxin transporter. The functional characterization of WAT1 as a tonoplast-localized auxin transporter in plants will provide insight into assigning a function to other members of the WAT1 family. Plant growth conditions and β-glucuronidase assays A. thaliana plants (Col-0) were used. The mutant lines wat1-1 and wat1-3 were isolated from a transfer DNA-mutagenized population as described [19] . For in vitro experiments, seeds were surface-sterilized and sown on agar-solidified MS medium including sucrose (10 g l −1 ) and MES buffer (0.5 g l −1 ) pH 5.7 in culture rooms with an 8-h photoperiod (120 μmol photons per m s −1 ) at 22 °C. Plants were also routinely grown in Jiffy peat pellets (9 h light, 200 μmol photons per m s −1 , 22 °C, 65% relative humidity). GUS assays on pro WAT1:GUS lines were conducted as described previously [47] . Briefly, tissues were incubated in 2 mM X-Gluc (5-bromo-4-chloro-3-indoxyl-β- D -glucuronic acid, Euromedex, Souffelweyersheim, France), 0.1% Triton X-100, 50 mM sodium phosphate buffer (pH 7.0) and 1 mM each of potassium ferri/ferrocyanide. After the reaction, the GUS staining was fixed for 1 h in 3% paraformaldehyde, 0.5% glutaraldehyde and 50 mM sodium phosphate buffer (pH 7.0). Microarray analysis Microarray analysis was performed with a 22-k CATMA Arabidopsis array. Two independent biological comparisons were carried out. RNA integrity check, cDNA synthesis, hybridization and array scanning were done as described [48] . Statistical analysis and identification of differentially expressed genes were done as described [49] . Expression data from this article were deposited according to MIAME (‘Minimum Information About a Microarray Experiment’) standards in the GEO (‘Gene Expression Omnibus’) database ( http://www.ncbi.nlm.nih.gov/geo ) under accession number GSE10716 and at CATdb (‘Complete Arabidopsis Transcriptome database’, http://www.urgv.evry.inra.fr/CATdb/ ) under the project name ‘RS06-04_Noduline-like’. Coexpression analysis was performed using the Arabidopsis Coexpression Data Mining Tools from the University of Leeds [21] . WAT1 cDNA cloning for expression in yeast WAT1 cDNA amplified from 10-day-old in vitro Arabidopsis Col-0 plantlets using N21-PstI/S (5′-AAAACTGCAGATGGCGGATAACACCGATAA-3′) and N21-SalI/AS (5′-ACGCGTCGACTCAAACATTGTCCGTTGACT-3′) primers was cloned into the pDR196 yeast expression vector. For subcellular localization, the GFP sequence was fused in carboxy terminal to WAT1 before cloning into pDR196 as well. 3 H-tryptophan and 3 H-IAA uptake assays in yeast Yeast cells were grown (OD 600 =1) in liquid minimal medium plus dextrose, collected by centrifugation (6,000 g , 5 min), washed (10 mM sodium citrate, pH 4.5) and resuspended (OD 600 =3) in 5 ml transport buffer (10 mM sodium citrate, 2 mM glucose, 20 mM ammonium sulphate, pH 4.5). Where appropriate, the buffer was supplemented with 500 μM of non-radiolabelled competitors. Uptake assays were initiated by adding L -[5- 3 H]tryptophan (20 Ci mmol −1 ; Hartmann Analytic, Oberhausbergen, France) or 3-[5(n)- 3 H]indolylacetic acid (20 Ci mmol −1 ; GE Healthcare, Ramonville Saint-Agne, France) to a final activity of 10.0 μCi ml −1 . At various time points, 500 μl of cell suspension were removed, filtered (Whatman GF/C) and washed (10 ml 10 mM sodium citrate, pH 4.5). Retained radioactivity was quantified (Packard-1900TR liquid scintillation analyser, Meriden, USA). Auxin uptake assays in oocytes The coding region of WAT1 was subcloned into a Gateway compatible vector (pGEMGWC) derived from the pGEMHE vector [50] . WAT1 cRNAs were transcribed from the WAT1 -pGEMGWC construct linearized with Sph I, using mMESSAGE mMACHINE T7 Ultra kit (Ambion). Oocytes preparation and injection (50 nl per oocyte) were performed as described [51] . Oocytes were injected with WAT1 cRNA (1 ng nl −1 ) or water only (control). Oocytes were kept for 2 days at 18 °C in ‘ND96 medium’ (96 mM NaCl, 2 mM KCl, 1.8 mM MgCl 2 , 1 mM CaCl 2 , 2.5 mM Na-pyruvate, 5 mM HEPES-NaOH pH 7.4) with 50 mg ml −1 gentamycin. For IAA uptake assays, oocytes were incubated 20 min in 1 ml of a modified ND96 medium (buffered to pH 6 with 5 mM MES-NaOH) containing 1 μM IAA (labelled with 100 nM 3 H-IAA). 14 C-IAA transport assays in Arabidopsis vacuoles Protoplasts and vacuoles were isolated as described [52] . Vacuole transport experiments were carried out using 0.1 μCi 14 C-IAA (20 μM) and 0.1 μCi 3 H 2 O to determine the vacuolar volume. 14 C-IAA (20 μM) was used to ensure sufficient vacuole loading. Transport experiments were performed using the silicon oil method at pH 7.2 as described [52] , [53] , either in the absence of NH 4 Cl and the presence of 4 mM Mg-ATP or in the presence of 5 mM NH 4 Cl without Mg-ATP to avoid the generation of an electrochemical gradient. Verification that auxin is not modified within the vacuole To analyse the identity of the 14 C radioactivity accumulated in the vacuoles after 18-min incubation time, HPLC fractionation was used. The analytical reversed-phase HPLC system included a Hypersil C18 ODS-2 (5 μm, 250 × 4.6 mm 2 ; Thermo Scientific) column, whereby a 30-min linear gradient of 10–48% methanol at a flow rate of 0.5 ml min −1 was used to separate the samples. The solutions of the mobile phase contained 0.01% H 3 PO 4 . Ultraviolet absorbance of IAA was monitored at a wavelength of 210 nm with a photodiode array detector (Dionex PDA-100). Authentic IAA (2 mM; Fluka 57330) was used as the reference compound. The upper aqueous phases (50 μl) of five vacuolar uptake reactions were pooled and mixed with 0.2 vol trichloroacetic acid 240 mg ml −1 and centrifuged at 12,000 g for 5 min at 4 °C. Two hundred microlitres of sample was loaded onto the C18 column and fractions were collected every minute, mixed with 3 ml Ultima Gold scintillation cocktail (PerkinElmer) and measured by liquid scintillation counting. Western blot Proteins were extracted (1% NP-40, 200 mM NaCl, 10 mM Tris–HCl pH 7.5, 5 mM EDTA, 10% glycerol, protease inhibitor cocktail, Roche, USA), separated on a 4% stacking and 12% separation SDS–PAGE gel and transferred to a polyvinylidene fluoride membrane (Millipore). The presence of particular proteins was detected using rabbit primary polyclonal antibodies (Agrisera, Sweden) raised against organelle-specific markers. Quantification of endogenous auxin metabolites in isolated vacuoles Vacuole isolation was performed as published [54] with minor modifications. Plants were grown for 60 days instead of 35 days, incubation with the protoplast enzyme solution was performed at 25 °C and neutral red starting concentration was 0.3% instead of 0.1%. Vacuole fractions (ca. 0.5 ml) were diluted five times with 1% acetic acid (v/v), extracted for 15 min and purified by solid phase extraction with the addition of the following internal standards: 5 pmol [ 13 C 6 ]IAA-Ala, [ 13 C 6 ]IAA-Asp, [ 13 C 6 ]IAA-Glu and [ 13 C 6 ]IAA-Leu; 10 pmol [ 13 C 6 ]ANT, [ 13 C 6 ]IAA, [ 13 C 6 ]IAM, [ 13 C 6 ]oxIAA and [ 2 H 2 ]TRA; 25 pmol [ 13 C 6 ]IAN and 50 pmol [ 2 H 5 ]TRP. Unlabelled and heavy labelled IAA and IAA metabolite standards were purchased or synthesized as described [55] . All samples were loaded onto Isolute C8 (EC) columns (500 mg per 3 ml; International Sorbent Technology, Hengoed, Mid Glamorgan, UK) pre-washed with methanol and 1% acetic acid in water (2 ml), washed with 10% methanol in 1% acetic acid (2 ml) and eluted with 70% of methanol acidified with 1% acetic acid (2 ml). The eluates were evaporated to dryness and dissolved in 20 μl of mobile phase before liquid chromatography–multiple reaction monitoring–mass spectrometry analysis using a 1290 Infinity LC system and a 6460 Triple Quad LC/MS system (Agilent Technologies, Santa Clara, USA) as described [55] . Localization of WAT1:GFP and BFA treatments For co-localization, F1 seeds obtained from crossings between p35S::WAT1:GFP , a line that fully restores the wat1 phenotype [19] , and plants expressing either YFP-VAM711, YFP-RabG3f or YFP-NPSN12 (ref. 29 ) were surface sterilized, stratified for 24 h and grown for 4 days under long-day conditions on half-strength MS plates (5% sucrose, 0.8% agar, pH 5.8). Before observation, seedlings were mounted in liquid half-strength medium (without sugar). Observation was carried out using a Leica DMIRE2 laser scanning confocal microscope. GFP and YFP were, respectively, excited with the 488-nm (GFP) and 514-nm (YFP) line of an Argon laser, and emission was detected between 500 and 530 nm for GFP and between 532 and 560 nm for YFP. For co-localization, the ‘Colocalization’ plugin for ImageJ was used with default settings. Four-day-old p35S::WAT1:GFP seedlings grown on half-strength MS were transferred to liquid medium containing dimethylsulphoxide (DMSO) as control or 50 μM BFA (Sigma-Aldrich). Seedlings were incubated in the dark for 3 h and transferred to fresh liquid medium containing 5 μM of the lipophilic dye FM4-64 (Invitrogen/Molecular Probes) for 5–15 min. Seedlings were rinsed once in MS medium and once in water before mounting them in water on microscope slides. For observation, a Zeiss Observer.Z1 LSM780 confocal microscope was used. GFP and FM4-64 were excited with a 488-nm Argon laser and emission was detected between 490 and 569 nm for GFP and between 668 and 757 nm for FM4-64. Local auxin applications Lanolin wax (Sigma) was melted at 50 °C before either 2,4- D or 1-NAA were added to a final concentration of 1 mM from 100 mM stocks in DMSO. For control treatments, lanolin was mixed with DMSO (1% final concentration). With the help of sterile wooden toothpicks, rings of wax were then applied onto the second internodes of 5-week-old plants. Plants were grown in long day, 16 h of light and 8 h of dark. Ten days after application internodes were collected, they were hand-sectioned at the site of application and stained in phloroglucinol (in 20% HCl) for 2 min. A Zeiss Axioplan 2 imaging system with a differential interference contrast (DIC) set-up was used for observation and capture of pictures. Accession codes: Expression data from this article were deposited according to MIAME standards in the GEO database under Accession code GSE10716 and at CATdb ( http://www.urgv.evry.inra.fr/CATdb/ ) under the project name RS06-04_Noduline-like. How to cite this article: Ranocha, P. et al . Arabidopsis WAT1 is a vacuolar auxin transport facilitator required for auxin homoeostasis. Nat. Commun. 4:2625 doi: 10.1038/ncomms3625 (2013).